Coherent control in a semiconductor optical amplifier operating at room temperature Quantum decoherence times in semiconductors are extremely short, particularly at room temperature where the quantum phase is completely erased in a fraction of a picosecond. However, they are still of finite duration during which the quantum phase is well defined and can be tailored. Recently, we demonstrated that quantum coherent phenomena can be easily accessed by examining the phase and amplitude of an optical pulse following propagation along a room temperature semiconductor optical amplifier. Taking the form of Rabi oscillations, these recent observations enabled to decipher the time evolution of the ensemble states. Here we demonstrate the Ramsey analogous experiment known as coherent control. Remarkably, coherent control occurs even under room temperature conditions and enables to directly resolve the dephasing times. These results may open a new way for the realization of room temperature semiconductor-based ultra-high speed quantum processors with all the advantages of upscaling and low-cost manufacturing. A Schrödinger wavefunction describing an isolated quantum two-level system of energy Δ E acquires a quantum phase, which is linear in time; Φ= Δ E·t/ħ , according to the time-evolution operator. In the presence of scattering and dephasing processes, as for an ensemble of states, the well-defined quantum phase is erased on timescales of the coherence time. A direct way to study the decay of the quantum phase is by imposing coherence at a known time instance and probing the temporal evolution of its dephasing. The class of measurements of this kind is known as coherent control where the outcome of the probing operation depends on the phase relation between the field and the quantum state. Coherent control has been demonstrated in a variety of quantum systems [1] , [2] , [3] , [4] , [5] . In semiconductors, however, tailoring the quantum interaction of the resonant interband transition is considered more challenging. Being a densely packed interacting atomic system, semiconductors exhibit extremely short coherence times of no more than a few hundreds of femtoseconds at room temperature. By operating at cryogenic temperatures, demonstrations of coherent control in semiconductors were revealed in structures of different dimensionalities using various methods. In the early report of Heberle et al. [6] , and also in refs 7 , 8 , 9 , interferometric four-wave mixing was used. Other methods such as upconversion optical sampling [10] , [11] , [12] , [13] and photoluminecense measurements [14] , [15] , [16] were also applied to demonstrate coherent control, as were photocurrent measurements [17] . To our best knowledge, no observations of Ramsey-type coherent control on the interband transition were reported to date in room temperature semiconductors. Moreover, coherent control of ensemble states along an active semiconductor waveguide poses further challenges, as in addition to the quantum interaction, cumulative effects related to propagation affect the observation. Recently, we demonstrated an experiment that enables to readily identify quantum coherent interactions taking place during the propagation of a short pulse in a semiconductor optical amplifier (SOA) even in the presence of significant room-temperature dephasing. The principle of the experiment was that the complex electromagnetic field (phase and amplitude) of the pulse was characterized at the SOA output with a temporal resolution of nearly a single femtosecond. This was demonstrated for the first time in a quantum wire-like (commonly referred as quantum dash) SOA [18] where systematic, coherent Rabi oscillations and self-induced transparency were clearly observed. Furthermore, by a comparison with a simulation of the Maxwell and Schrödinger equations [19] , we were able to decipher the time evolution of effective ensemble states along the propagation axis. Following the demonstrations of Rabi oscillations in a quantum dash amplifier [18] , the observations were repeated in zero-dimensional quantum systems, as reported for an InP based quantum dot SOA operating at 1,550 nm (ref. 20 ) and in a 1,300-nm GaAs quantum dot amplifier [21] . Using the high-resolution technique demonstrated in refs 18 , 20 , we turn in the present work to show coherent control of ensemble states along a SOA. This is shown by sending pairs of optical pulses separated by a known time interval and measuring the coherent signatures imprinted on the second (trailing) pulse. Surprisingly, these are observed even under room temperature conditions and in the presence of an inhomogeneously broadened gain medium. The experimental setup constructed here is in fact a pump–probe system that exhibits an extremely high, sub-optical-cycle resolution, which is orders of magnitude finer than conventional pump–probe systems. Therefore, it is capable of operating in the fully quantum coherent regime. The experiments carried out are analogous to the Ramsey experiment and enable to resolve directly the quantum dephasing times. Equivalently, they can also be analysed in the frequency domain where the interaction between the pump, the delayed probe and the nonlinear medium yields a degenerate four-wave-mixing-like interaction [22] . Device characteristics and experimental conditions The active gain section of the SOA consisted of four, molecular beam epitaxy grown, InAs quantum dots layers each five monolayers thick, separated by 20 nm In 0.825 Al 0.238 Ga 0.234 As barriers. Low-temperature photoluminescence spectra of the quantum dot material exhibiting an optical transition at the energy of 0.79 eV and a full width at half maximum inhomogeneous line broadening of 31 meV are presented in Fig. 1a . The room-temperature light versus current ( L – I ) curve of the fully processed SOA and the corresponding electroluminescence spectra are presented in Fig. 1b . The lower inset of the figure shows schematically the energy band diagram of the complete epitaxial structure. The experiments for which the results are reported were performed at a drive current density of 500 A cm −2 where the device is absorbing. The optical pulses were generated by an optical parametric oscillator (OPO) and characterized using the frequency-resolved optical gating (FROG) system. The time domain electromagnetic field of the optical pulses used for the experiments is presented in Fig. 1c . The time-dependent electrical field, E(t) , is represented by the intensity envelope, I(t); E(t)=√I(t) exp −iφ(t) with the instantaneous frequency (chirp), ν(t) , being the time derivative of the phase, φ(t) : ν(t) =−( 1/2π )( dφ/dt) . The pulses were spectrally located at 1,530 nm and had a full width at half maximum duration of 150 fs. More details of the sample and the experimental conditions are described in the Methods section. 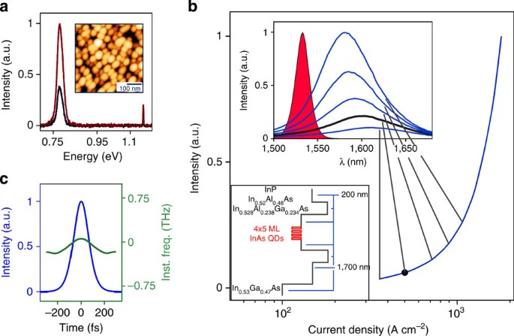Figure 1: Device characteristics and experimental conditions. (a) Photoluminescence spectra of the quantum dot layer at 10 K for excitation powers of 10 W cm−2(dark blue) and 21 W cm−2(red). Inset presents atomic force microscopy image (AFM). (b) Room-temperatureL–Icharacteristics and electroluminescence spectra of the fully processed amplifier. The black dot on theL–Icurve represents the operation point chosen for the experiments with the corresponding spectrum shown in a thick black line. The lower inset shows the schematic energy band diagram. (c) Time-dependent intensity and instantaneous frequency profiles of the reference pulse. The profiles are presented after removal of the time ambiguity resulting from the second harmonic generation (SHG) FROG characterization scheme. Figure 1: Device characteristics and experimental conditions. ( a ) Photoluminescence spectra of the quantum dot layer at 10 K for excitation powers of 10 W cm −2 (dark blue) and 21 W cm −2 (red). Inset presents atomic force microscopy image (AFM). ( b ) Room-temperature L–I characteristics and electroluminescence spectra of the fully processed amplifier. The black dot on the L–I curve represents the operation point chosen for the experiments with the corresponding spectrum shown in a thick black line. The lower inset shows the schematic energy band diagram. ( c ) Time-dependent intensity and instantaneous frequency profiles of the reference pulse. The profiles are presented after removal of the time ambiguity resulting from the second harmonic generation (SHG) FROG characterization scheme. Full size image Experimental setup and measured results The origin of the high temporal resolution of the pump–probe experiment reported in this paper stems from the fact that the actual field is measured rather than the transmission of the probe pulse. This is achieved by using the cross-correlation FROG (X-FROG) technique [23] . A schematic of the experimental arrangement is depicted in Fig. 2 . The 150-fs pulses emitted by the OPO were split to form two identical pump and probe pulses separated by a predetermined delay, Δ τ . The two pulses were coupled to the quantum dot SOA, at the output of which the complex electromagnetic field of both pulses was retrieved from the X-FROG measurement with a temporal resolution of nearly 1 fs. 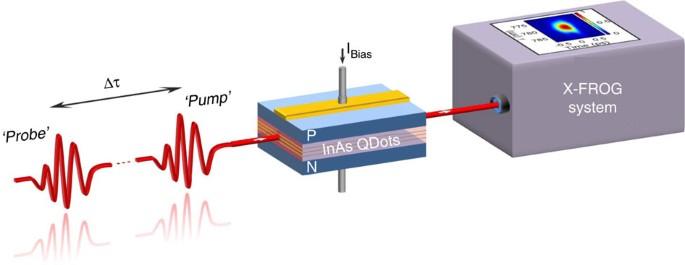Figure 2: Pump–probe–FROG characterization setup. Short pulses emitted from an OPO were split into phase-locked pump and probe pulses. After propagating through the InAs quantum dot semiconductor medium, the complete optical field was measured using the X-FROG scheme. The experiments were carried out at room temperature. Figure 2: Pump–probe–FROG characterization setup. Short pulses emitted from an OPO were split into phase-locked pump and probe pulses. After propagating through the InAs quantum dot semiconductor medium, the complete optical field was measured using the X-FROG scheme. The experiments were carried out at room temperature. Full size image The measured optical fields of the pump and probe pulses are presented in Fig. 3 . For very short pump–probe delays, the tails of the pump and probe pulses overlap and interfere linearly. This interference, occurring in the presence of the resonant medium, masks any signature of the coherent interaction and therefore short delays are avoided. For a delay of 500 fs or more, the overlap is sufficiently small to be negligible; hence, we examine traces having a nominal pump–probe delay of 500 fs and longer. 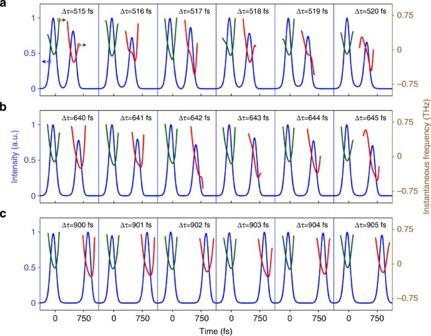Figure 3: Measured electromagnetic field. The amplitude (blue traces) and instantaneous frequency (chirp) profiles (green: pump; red: probe) for nominal delays of (a) 515 (b) 640 and (c) 900 fs as measured by the X-FROG system. Instantaneous frequency traces are measured relative to the carrier frequency. Probe pulses are delayed by 1 fs consecutively. In all traces and all nominal delays, the pump pulses exhibit similar parabolic signatures. When probe pulses arrive close to the pump, coherent signatures are observed. When the probe pulses arrive at long nominal delays, coherent signatures cease to appear. Intensity profiles are normalized to unity at their peak. Figure 3: Measured electromagnetic field. The amplitude (blue traces) and instantaneous frequency (chirp) profiles (green: pump; red: probe) for nominal delays of ( a ) 515 ( b ) 640 and ( c ) 900 fs as measured by the X-FROG system. Instantaneous frequency traces are measured relative to the carrier frequency. Probe pulses are delayed by 1 fs consecutively. In all traces and all nominal delays, the pump pulses exhibit similar parabolic signatures. When probe pulses arrive close to the pump, coherent signatures are observed. When the probe pulses arrive at long nominal delays, coherent signatures cease to appear. Intensity profiles are normalized to unity at their peak. Full size image The experiments are performed so that we first select a nominal delay, Δ τ , and then scan it in 1 fs steps (which is about one fifth of an optical cycle). For each step, the amplitude and chirp profiles for both pulses are acquired. Exemplary results are shown in Fig. 3a–c for nominal Δ τ values of 515, 640 and 900 fs, respectively. The amplitude and instantaneous frequency profiles of all leading pump pulses arriving at t =0 are identical, as the semiconductor fully decoheres during the time between subsequent pulse pairs. The parabolic chirp profile of the leading pump pulses is a well-known signature of the interaction stemming from a modulation of the refractive index by the excitation of carriers under absorbing conditions [18] , [24] , [25] . The modulation of the refractive index by the excited population plays a dominant role in understanding the traces obtained by the X-FROG system and is the source of the high sensitivity to the state of the quantum ensemble [18] . When the pump pulse arrives, all quantum states comprising the ensembles are well averaged over the Bloch state space, and hence all pump pulses interact in an identical manner. In contrast, the probe pulses exhibit a fundamentally different behaviour. Although their amplitude profiles are preserved as the delay is scanned, the instantaneous frequency profiles change considerably for every delay step as seen in Fig. 3a for the nominal delay of 515 fs. The figure shows, for example, that a probe pulse arriving at a delay of 515 fs experiences a valley-like chirp profile similar to that of the pump. However, the phase change associated with a delay that is merely 1 fs longer yields a completely different chirp profile. Further tuning of the delay results in a continuous variation of the probe chirp profile. Recalling that the evolution of the quantum states is imprinted on the phase of the electromagnetic field, and hence on the chirp profile [18] , means that for every delay the probe pulse interacts differently with the ensemble of quantum systems comprising the medium. As the probe pulse is further delayed and the chirp profile continues to vary, a point may be reached where the probe chirp profile can actually change its nature. This is observed in Fig. 3a for the delay of 520 fs where the instantaneous frequency initially increases instead of decreasing, suggesting that the leading edge of the probe pulse actually undergoes an amplification process rather than absorption. The fact that the pump pulse always experiences the same parabolic chirp behaviour while the chirp profile of the probe depends on its arrival time implies that the pump pulse locks the phases of the quantum states comprising the ensemble (as predicted in ref. 19 ), which otherwise would have been spread randomly over a 2 π range. Once the quantum phases of the ensembles are aligned and well defined, time-keeping becomes possible so that the arrival time of the probe pulse plays a role in determining the outcome of the interaction. Figure 3a presents only a subset of six traces around the delay of 515 fs, but the optical fields behave in the same manner at longer delays. This behaviour persists of course as long as the quantum states along the amplifier have not decohered. For longer nominal delays, the quantum states comprising the ensemble start to dephase and gradually the coherent imprints diminish. Therefore, the experimental system is capable of measuring directly the evolution of the dephasing process and to determine the time, following the pump perturbation, at which the quantum coherence ceases to exist. Figure 3b illustrates the results measured when the probe is nominally delayed by 640 fs. This subset of measurements shows that clear coherent signatures are still observable; however, they are less pronounced compared with the traces in Fig. 3a . As the probe pulse is further delayed to a nominal delay of 900 fs, the coherent signatures disappear completely and the profiles of both pump and probe pulses are similar in nature exhibiting a parabolic form independent of the delay. This means that the quantum states have fully dephased and that the electromagnetic field of the second probe pulse interacts with the semiconductor in a similar manner to that of the first pulse. Therefore, these experiments constitute a direct measurement of the quantum dephasing. In Fig. 3a,b , the evolution of the relative probe intensities are seen to vary. These variations may be due to propagation effects (combining two photon absorption and linear dispersion) or possibly even a coherent two-photon Ramsey interaction. For practical reasons, the experiments were performed at a single wavelength, which was on the high energy side of the absorption peak. It is expected that for larger absorption, the observed phenomena can be enhanced but the signal-to-noise ratio would deteriorate. To obtain a physically meaningful figure of merit for the decoherence time, we estimate the time that the quantum states have been given to dephase without the presence of the electromagnetic field, which serves as an aligning potential. Limiting the field to a level of 1% of the pulse peak intensity, results in a dephasing time ranging from 360 to 390 fs for the room-temperature semiconductor under the specific bias conditions chosen here. The figure of merit, extracted from the coherent control experiment, is similar to coherence times obtained from transient four-wave-mixing measurements in a room-temperature GaAs SOA [26] and from temperature-dependent photoluminescence measurements of a single quantum dot [27] . The physical origin of the decoherence is mainly incoherent thermalization of carriers from the high-energy reservoir. Under the absorption conditions used here, the reservoir population is moderate and hence relaxation into the quantum dots is mediated mainly by phonon scattering while carrier–carrier scattering is negligible. Numerical calculation The experimental results can be modelled qualitatively considering that the SOA behaves as an effective ensemble of two-level systems. Describing the semiconductor medium as sequentially placed two-level systems, which are fed incoherently from a carrier reservoir, has been used to describe propagation of short pulses along a quantum cascade laser [28] and in inhomogeneously broadened self-assembled quantum dashes [18] and quantum dots [20] . The model calculates the coevolution of the electromagnetic field and the electronic wavefunctions along the propagation axis according to the coupled Maxwell and Schrödinger equations for every time iteration using the density matrix formalism (see ref. 19 ). A key aspect of the model is the inclusion of the carrier density dependence of the refractive index. Therefore, self-phase modulation appears inherently in the simulation. A more quantitative description requires inclusion of the inhomogeneous broadening and other propagation effects, notably distributed two photon and free carrier absorption, as well as linear dispersion. The simulation results therefore describe the experiments on a qualitative basis, as in refs 18 , 20 . A calculated example describing the interaction along the propagation axis at an arbitrary iteration step of the simulation is shown in Fig. 4a . The figure shows the intensity of the pulses together with the spatially dependent population inversion of the effective two-level system, ρ 11 − ρ 22 , where ρ 11 and ρ 22 denote the probability amplitudes of the excited and ground states, respectively, and are the diagonal elements of the density matrix. In Fig. 4a , we plot the calculated interaction for two different pump–probe delay intervals, 500 and 502 fs, which correspond to a phase difference of almost π in the optical field. As in the experiment, the simulation was prepared so that the gain medium is initially in the absorbing regime where the population inversion is negative and the quantum state having no predetermined phase. For both delay values, the pump pulse undergoes an absorption process, which increases the population inversion. The probe arriving at a delay of 500 fs experiences a fully absorptive process (with the population inversion continuously increasing). However, the probe pulse arriving 2 fs later, at 502 fs, experiences an amplification process on its leading edge (with the population inversion decreasing), which turns into an absorption process for the rest of the pulse duration. This initial gain process results in the pulse intensity profiles shown in Fig. 4b . As the index of refraction is related to the excited carrier populations, the two cases of absorption and gain mark complimentary signatures in the resultant chirp of the optical field. 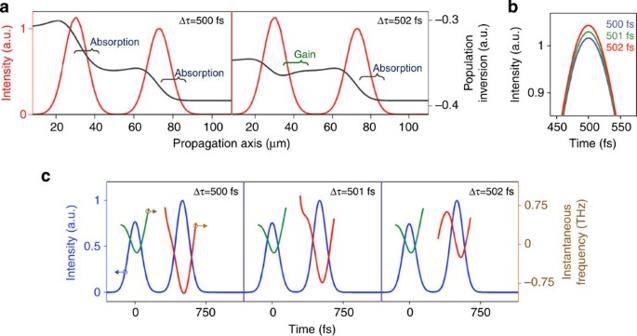Figure 4: Numerical calculation. (a) Calculated example of the intensity (red) and population inversion of the effective two-level system (black) along the propagation axis for two pump–probe delays around a nominal delay of 500 fs. For 500 fs, both pulses undergo absorption, while, when the probe pulse is delayed to 502 fs, the leading edge of the probe pulse initially experiences amplification. (b) Probe pulse intensities in the vicinity of the peak for delays of 500 (blue), 501 (green) and 502 fs (red) showing the effect of the gain on the probe amplitudes. (c) Calculated intensity (blue) and instantaneous frequency (green: pump; red: probe). The pump pulse experiences a consistent parabolic chirp profile, while the signature imprinted on the instantaneous frequency of the probe is modified significantly as the pump–probe delay is changed in steps of 1 fs. The occurrence of an amplification or absorption process inaresults in a corresponding increase or decrease of the chirp profile in the pulse leading edge inc. Figure 4: Numerical calculation. ( a ) Calculated example of the intensity (red) and population inversion of the effective two-level system (black) along the propagation axis for two pump–probe delays around a nominal delay of 500 fs. For 500 fs, both pulses undergo absorption, while, when the probe pulse is delayed to 502 fs, the leading edge of the probe pulse initially experiences amplification. ( b ) Probe pulse intensities in the vicinity of the peak for delays of 500 (blue), 501 (green) and 502 fs (red) showing the effect of the gain on the probe amplitudes. ( c ) Calculated intensity (blue) and instantaneous frequency (green: pump; red: probe). The pump pulse experiences a consistent parabolic chirp profile, while the signature imprinted on the instantaneous frequency of the probe is modified significantly as the pump–probe delay is changed in steps of 1 fs. The occurrence of an amplification or absorption process in a results in a corresponding increase or decrease of the chirp profile in the pulse leading edge in c . Full size image Calculated amplitude and chirp temporal profiles of the output pulses are shown in Fig. 4c for three consecutive probe arrival times. All pump pulses are identical and exhibit the parabolic profile, similar to the ones measured experimentally. The two delay intervals, Δ τ =500 and 502 fs yield a complimentary chirp profile on the leading edge of the probe pulse corresponding to either gain or absorption, consistent with the experimental results of Fig. 3a . The calculated response, which shows the initial process of amplification (at Δ τ =502 fs), resembles the measured chirp profile for a delay of Δ τ =520 fs. As in the experimental results, the simulations reveal that when the probe pulse is further delayed, the coherent features decay and eventually vanish. However, a proper quantitative description of the dephasing process requires invoking the inhomogeneous broadened version of the Maxwell–Schrödinger model [20] . To obtain an intuitive understanding of the interaction, we analyse it using the geometrical representation of the Bloch sphere. Although in the experiment, propagation effects may cause a longitudinal variation of the pulse, which quantitatively changes the details of the observation, the principal behaviour remains intact. It is therefore found helpful to describe the experiments using the geometrical representation. We use the notation of ref. 29 to represent the state vector, , and the field vector, ; hence, the equation of interaction follows the form of the precession of a classical gyromagnet in a magnetic field: When the interaction occurs resonantly and the relationship between the quantum phase and the field phase is preserved, the field vector takes on the form: meaning that it spans the x – y plane. In equation (2), Ω stands for the Rabi frequency and φ 0 is the angle of the field vector in the x – y plane. The important thing to realize in this intuitive picture is that the angle φ 0 depends on the absolute phase of the optical field so that the probe field vector exhibits an angle φ 0 , which is larger by ω 0 ·Δ τ compared with the pump field vector with ω 0 being the angular carrier frequency of the optical field (and equals Δ E/ħ on resonance) and Δ τ is once more the arrival time of the probe relative to the pump. 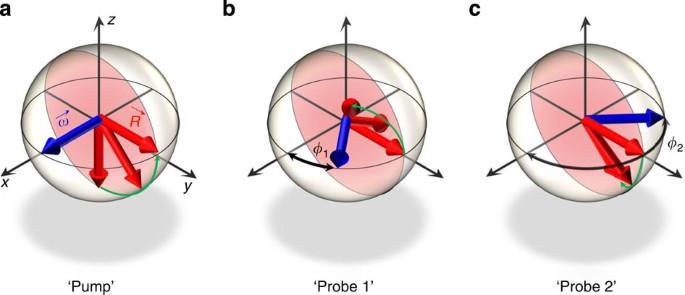Figure 5: Geometrical representation on the Bloch sphere. Field vectors are represented by blue arrows and state vectors are represented by red arrows. TheX,YandZcomponents of the state vector correspond to the real and imaginary parts of the coherence term of the density matrix,ρ12, and to the population inversion,ρ11−ρ22, respectively. In the example shown, the field vectors reside in thex–yplane. The delay at which the probe pulses arrive determines their orientation. (a) Pump pulses initiate the state vector to an intermediate state. (b) Probe arriving at a delay time corresponding to an angleφ1, which results in the ascending of the state vector (absorption). (c) Probe arriving at a later delay time corresponding to a larger angle ofφ2, which results in the descending of the state vector (amplification). A rotation ofπof the field vector requires a delay of half optical cycle, which is ~2.5 fs in this experiment. Figure 5 illustrates the geometrical representation of the interaction. The pump field vector arriving at t =0 is aligned along the x axis ( Fig. 5a ) and as a result of the interaction, the state vector evolves to some intermediate state for instance in the x – y plane as illustrated. Two probe pulses arriving at two different times correspond to two field vectors having different angles φ 1 and φ 2 . These field vectors cause the state vector to evolve either to the higher energy state or to the lower energy state, depending on their position relative to the state vector according to equation (1) as shown in Fig. 5b,c . A complimentary evolution is initiated, based on equation (2), if the two probe vectors are exactly at an angle of π relative to each other. At the wavelength we operate, 1,530 nm, the optical cycle is ~5 fs so that a π phase shift requires a delay of ~2.5 fs. This is the origin of the sensitivity of the outcome to delay variations of merely 1 fs. Figure 5: Geometrical representation on the Bloch sphere. Field vectors are represented by blue arrows and state vectors are represented by red arrows. The X , Y and Z components of the state vector correspond to the real and imaginary parts of the coherence term of the density matrix, ρ 12 , and to the population inversion, ρ 11 − ρ 22 , respectively. In the example shown, the field vectors reside in the x – y plane. The delay at which the probe pulses arrive determines their orientation. ( a ) Pump pulses initiate the state vector to an intermediate state. ( b ) Probe arriving at a delay time corresponding to an angle φ 1 , which results in the ascending of the state vector (absorption). ( c ) Probe arriving at a later delay time corresponding to a larger angle of φ 2 , which results in the descending of the state vector (amplification). A rotation of π of the field vector requires a delay of half optical cycle, which is ~2.5 fs in this experiment. Full size image To summarize, in this study we have used a unique pump–probe–FROG system that exhibits very high time resolution and hence avails measurements in the coherent regime. The system enabled to demonstrate that the outcome of the light–matter interaction in an electrically driven SOA operating at room temperature is sensitive to the quantum phase as long as it has not decohered. At the same time, new details of the behaviour of the quantum ensemble were disclosed and the dephasing time was quantified directly. These experiments mark another step in obtaining control over coherent quantum effects in practical semiconductor devices, which may lead to the demonstration of additional coherent effects (for example, photon echoes) and eventually to the implementation of an ultra-high-speed quantum processor based on the scalable low-cost semiconductor technology. Experiment details One hundred and fifty-femtosecond-wide pulses were generated by a tunable OPO (Spectra-Physics OPAL) with a repetition rate of 82 MHz. The OPO output was split to form two identical pulses with a controlled delay between them, each having an average power of 3 mW at the amplifier input. For pulse characterization, we employed a home-built X-FROG system. A reference pulse, extracted from the pulsed oscillator, gated both pulses at the output of the SOA on a 0.5-mm long LiNbO 3 type-1 nonlinear crystal to generate the sum-frequency signal required for the X-FROG scheme. The complex envelopes (phase and amplitude) of the electromagnetic field of both pulses were obtained using the conventional phase retrieval method of the FROG technique, resulting in typical convergence errors below 0.004. The temporal resolution of the X-FROG system as well as of the delay line in the Ramsey analogous set up was ~0.1 fs, well below one optical cycle. These resolutions are determined by the DC motors driving the two delay lines. Spectral marginal were used for improved accuracy and removal of systematic errors. Quantum dot amplifier The 1.5-mm-long quantum dot SOA comprises an active region with four InAs dot layers grown by molecular beam epitaxy, each formed by a nominal deposition of five InAs monolayers with the layers separated by 20 nm In 0.528 Al 0.238 Ga 0.234 barriers. The N-doped substrate serves as the cladding layer. The 200-nm InP layer (inset of Fig. 1b ) was grown so as to improve the surface quality. The rather wide 200 nm InAlGaAs confinement region grown on each side of the quantum dots region led to long carrier transport times. The density of the quantum dots was about 5 × 10 10 cm −2 , with a typical base dimension of 20 nm by 3–4 nm and a height of 3–4 nm. Lateral confinement was achieved by a 3-μm-wide ridge waveguide and the amplifier length was 1.5 mm. The gain peak was spectrally located at 1,580 nm and the bandwidth at 10% below the peak was 150 nm. The homogeneous linewidth at room temperature was estimated to be ~3.75 meV. Experiments have shown that both adjacent quantum dots and neighbouring dot layers are quantum mechanically decoupled [30] . Two layer dielectric anti-reflection coatings were applied on the end facets of the waveguide. Under the bias current density of 500 A cm −2 , the propagated pulses maintained their short durations. How to cite this article: Capua, A. et al. Coherent control in a semiconductor optical amplifier operating at room temperature. Nat. Commun. 5:5025 doi: 10.1038/ncomms6025 (2014).